Investigation of exotic stable calcium carbides using theory and experiment It is well known that pressure causes profound changes in the properties of atoms and chemical bonding, leading to the formation of many unusual materials. Here we systematically explore all stable calcium carbides at pressures from ambient to 100 GPa using variable-composition evolutionary structure predictions using the USPEX code. We find that Ca 5 C 2 , Ca 2 C, Ca 3 C 2 , CaC, Ca 2 C 3 and CaC 2 have stability fields on the phase diagram. Among these, Ca 2 C and Ca 2 C 3 are successfully synthesized for the first time via high-pressure experiments with excellent structural correspondence to theoretical predictions. Of particular significance is the base-centred monoclinic phase (space group C 2 /m ) of Ca 2 C, a quasi-two-dimensional metal with layers of negatively charged calcium atoms, and the primitive monoclinic phase (space group P 2 1 /c ) of CaC with zigzag C 4 groups. Interestingly, strong interstitial charge localization is found in the structure of R -3 m -Ca 5 C 2 with semi-metallic behaviour. Unexpected chemical reactions can happen under extreme conditions, with emergence of rich phase diagrams and materials possessing intriguing properties. Recently, by combining variable-composition structure prediction methods with first-principles total energy calculations [1] , pressure-composition ( P-x ) phase diagrams were predicted for such binary systems as Mg-O (ref. 2 ) and Na-Cl (ref. 3 ). In both cases, the predicted unexpected compounds have been successfully synthesized [3] , [4] . Elemental carbon and calcium both exhibit rich diversity of stable and metastable phases under pressure [5] , [6] , [7] . Compressed calcium shows unique structural and electronic properties and exhibits the highest recorded superconducting critical temperature among pure elements [8] . For carbon, only graphite and diamond are experimentally known as thermodynamically stable solids (graphite is thermodynamically stable at ambient condition and diamond under high pressure), although numerous metastable phases are known. For example, by applying pressure to graphite at low temperatures, a new superhard carbon allotrope was found, and its properties match those of one of the theoretically predicted structures (M-carbon) [9] , [10] , [11] , [12] . For the Ca-C system, the well-known Ca carbides include CaC 2 and CaC 6 , whose high-pressure behaviours have been studied experimentally [13] , [14] , [15] and by ab initio calculations [16] , [17] , [18] , [19] , [20] . An interesting structural evolution has been uncovered under pressure: carbon atoms polymerize from dumbbells to one-dimensional (1D) chains to ribbons to two-dimensional (2D) graphene sheets in compressed CaC 2 (ref. 16 ) and from graphite sheets to a mixed sp 2 – sp 3 structure in CaC 6 (ref. 20 ). In addition, superconductivity was predicted in metallic high-pressure phases of CaC 2 with critical temperatures comparable to those observed in CaC 6 (ref. 16 ). Here, using variable-composition structure prediction code USPEX [1] , [9] , [21] , the pressure-composition phase diagram of the Ca-C system was explored in order to fully understand the structural diversity and evolution of the C–C bonding types under high pressure. This resulted in five newly predicted stable stoichiometries (Ca 5 C 2 , Ca 2 C, Ca 3 C 2 , CaC and Ca 2 C 3 ) with diverse carbon arrangements: isolated atoms in Ca 2 C, hitherto unknown zigzag tetramers in CaC, and ribbons consisting of five-membered rings in CaC 2 . Two phases (Ca 2 C and Ca 2 C 3 ) were confirmed experimentally via in situ synchrotron powder X-ray diffraction (PXRD) measurements. Most surprising is that the low-pressure phase (monoclinic C 2 /m structure) of Ca 2 C exhibits quasi-2D metallic behaviour and contains negatively charged calcium atoms. In addition, strong interstitial electron localization was found in the newly predicted R -3 m phase of Ca 5 C 2 , just as in compressed elements Li (ref. 22 ), Na (ref. 23 ) and Ca (ref. 6 ), as well as in the compound Mg 3 O 2 (ref. 2 ). Convex hull We have used the ab initio evolutionary algorithm USPEX [1] , [9] , [21] , which can simultaneously find stable stoichiometries and the corresponding structures in multicomponent systems, to explore stable Ca-C compounds and their structures. In these calculations, all stoichiometries were allowed (with the constraint that the total number of atoms in the unit cell be below 16 atoms), and calculations were performed at 10, 20, 40, 80 and 100 GPa. The pressure-composition phase diagram of the Ca-C system is given in Fig. 1a , in which the convex hull was obtained from the calculated enthalpies of the most stable structures for each composition at a given pressure. Thermodynamically, the convex hull at a given pressure connects the phases that are stable against decomposition into other binaries or the elements. 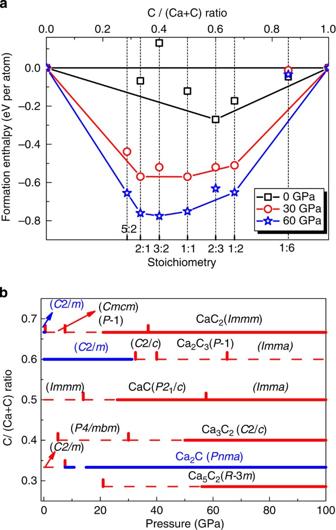Figure 1: Stability of new calcium carbides. (a) Convex hull diagram for the Ca-C system at selected pressures. At a given pressure, the compounds located on the convex hull are thermodynamic stable. (b) Pressure-composition phase diagram of the Ca-C system. Thick solid lines represent thermodynamically stable phases and dashed lines represent metastable phases (Red lines represent metal and blue semiconductor). Figure 1: Stability of new calcium carbides. ( a ) Convex hull diagram for the Ca-C system at selected pressures. At a given pressure, the compounds located on the convex hull are thermodynamic stable. ( b ) Pressure-composition phase diagram of the Ca-C system. Thick solid lines represent thermodynamically stable phases and dashed lines represent metastable phases (Red lines represent metal and blue semiconductor). Full size image Thermodynamically stable or metastable phases Using variable-composition evolutionary searches, we found that Ca 5 C 2 , Ca 2 C, Ca 3 C 2 , CaC, Ca 2 C 3 and CaC 2 have thermodynamic stability fields on the phase diagram: Ca 2 C 3 , stable from 0 to 28 GPa; Ca 5 C 2 , stable above 58 GPa; Ca 2 C, stable above 14 GPa; Ca 3 C 2 , stable from ∼ 50 GPa; CaC, stable above 26 GPa; and CaC 2 , stable above 21 GPa (see Figs 1b and 2 ). All crystallographic parameters are listed in Supplementary Table 1 . For all the newly predicted structures, calculated phonon dispersion relations confirmed their dynamical stability (see Supplementary Figs 1–5 and Supplementary Note 1 ). Surprisingly, our theoretical calculations show that the known phases of CaC 2 and CaC 6 are thermodynamically metastable at normal conditions (see Fig. 1a ); CaC 2 is thermodynamically stable only above 21 GPa, and CaC 6 does not have a thermodynamic stability field (BaC 6 is thermodynamically stable in the Ba-C system at 1 atm (ref. 24 )). We also explored metastable phases of Ca 2 C and CaC at lower pressure. The most stable low-pressure phase obtained for Ca 2 C has C 2 /m symmetry and that of CaC has Immm symmetry. The dynamical stability of these two thermodynamically metastable phases was confirmed via phonon calculations ( Supplementary Figs 6 and 7 ). 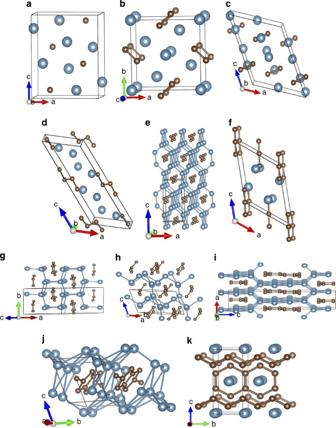Figure 2: The predicted crystal structures of stable Ca-C compounds. (a) Thermodynamically stablePnmastructure of Ca2C. (b) The metastable low pressureP4/mbmstructure of Ca3C2. (c) Thermodynamiclly stable high pressureC2/cstructure of Ca3C2. (d) Thermodynamically stableP21/cstructure of CaC. (e) Thermodynamically stable high pressureImmastructure of CaC. (f) Ca2C3crystallizes inC2/mstructure at pressures up to 28 GPa. (g) Thermodynamically metastableC2/cstructure of Ca2C3. (h) Thermodynamically metastableP-1 structure of Ca2C3. (i) Thermodynamically metastable high pressureImmaof Ca2C3. (j) Thermodynamically stableP-1 structure of CaC2. (k) Thermodynamically stableImmmstructure of CaC2. The blue and brown spheres represent calcium and carbon atoms, respectively. Figure 2: The predicted crystal structures of stable Ca-C compounds. ( a ) Thermodynamically stable Pnma structure of Ca 2 C. ( b ) The metastable low pressure P 4/ mbm structure of Ca 3 C 2 . ( c ) Thermodynamiclly stable high pressure C 2/ c structure of Ca 3 C 2 . ( d ) Thermodynamically stable P 2 1 / c structure of CaC. ( e ) Thermodynamically stable high pressure Imma structure of CaC. ( f ) Ca 2 C 3 crystallizes in C 2/ m structure at pressures up to 28 GPa. ( g ) Thermodynamically metastable C 2/ c structure of Ca 2 C 3 . ( h ) Thermodynamically metastable P -1 structure of Ca 2 C 3 . ( i ) Thermodynamically metastable high pressure Imma of Ca 2 C 3 . ( j ) Thermodynamically stable P -1 structure of CaC 2 . ( k ) Thermodynamically stable Immm structure of CaC 2 . The blue and brown spheres represent calcium and carbon atoms, respectively. Full size image In order to analyse these predicted structures, we recall that the C–C bond length depends on the bond order, and at 1 atm these lengths are 1.20 Å for the triple C–C bond, 1.33 Å for double bond and 1.54 Å for single C–C bond. The carbon patterns predicted for calcium carbides, on the basis of calculations presented in this work, are plotted in Fig. 3 . The carbon patterns together with their pressure range of existence in calcium carbides are summarized in Fig. 4 and in Supplementary Table 2 . Combining this knowledge with the results of Bader analysis (see Supplementary Table 1 ), we unravel very diverse chemistry. From the results of the Bader analysis, one can clearly see the correlation between the charge and volume: negatively charged calcium atoms occupy significantly greater volume. In addition, we observe the decrease in C–C bond order from triple to double to single bonds as pressure increases. Note, however, that at pressures up to 100 GPa, the carbon-richest stable compound is CaC 2 . Below we consider the predicted phases in order of increasing carbon content. 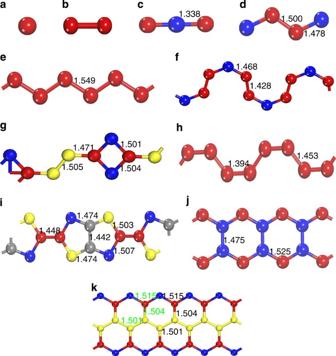Figure 3: Carbon patterns in the Ca-C system. (a) The isolated carbon anions in thePnmastructure of Ca2C. (b) Carbon dimers observed in theC2/mstructure of Ca2C,P4/mbmandC2/cstructures of Ca3C2,Immmstructure of CaC, andC2/morC2/cstructures of CaC2. (c) The carbon trimer occurs in theC2/mstructure of Ca2C3at zero pressure. (d) Zigzag C4groups observed inP21/cstructure of CaC at 20 GPa. (e) Zigzag carbon chains in theImmastructure of CaC at 58 GPa. (f) Carbon chains with two types of carbon-carbon bondings inC2/cstructure of Ca2C3at 34.5 GPa. (g) Carbon chains with four types of carbon-carbon bongdings inP-1 structure of Ca2C3at 40 GPa. (h) Armchair carbon chains in theCmcmstructure of CaC2at 4 GPa. (i) Carbon stripes in theP-1 structure of CaC2at 20 GPa. (j) Carbon ribbons in theImmmstructure of CaC2at 10 GPa. (k) Carbon ribbons in theImmastructure of Ca2C3at 65 GPa. Bond lengths (in Å) are given. The inequivalent C1, C2, C3, and C4 (occupying different Wyckoff positions in the unit cell, seeSupplementary Table 1) are shown by red, blue, yellow, and grey spheres, respectively. Figure 3: Carbon patterns in the Ca-C system. ( a ) The isolated carbon anions in the Pnma structure of Ca 2 C. ( b ) Carbon dimers observed in the C 2/ m structure of Ca 2 C, P 4/ mbm and C 2/ c structures of Ca 3 C 2 , Immm structure of CaC, and C 2/ m or C 2/ c structures of CaC 2 . ( c ) The carbon trimer occurs in the C 2/ m structure of Ca 2 C 3 at zero pressure. ( d ) Zigzag C 4 groups observed in P 2 1 / c structure of CaC at 20 GPa. ( e ) Zigzag carbon chains in the Imma structure of CaC at 58 GPa. ( f ) Carbon chains with two types of carbon-carbon bondings in C 2/ c structure of Ca 2 C 3 at 34.5 GPa. ( g ) Carbon chains with four types of carbon-carbon bongdings in P -1 structure of Ca 2 C 3 at 40 GPa. ( h ) Armchair carbon chains in the Cmcm structure of CaC 2 at 4 GPa. ( i ) Carbon stripes in the P -1 structure of CaC 2 at 20 GPa. ( j ) Carbon ribbons in the Immm structure of CaC 2 at 10 GPa. ( k ) Carbon ribbons in the Imma structure of Ca 2 C 3 at 65 GPa. Bond lengths (in Å) are given. The inequivalent C1, C2, C3, and C4 (occupying different Wyckoff positions in the unit cell, see Supplementary Table 1 ) are shown by red, blue, yellow, and grey spheres, respectively. 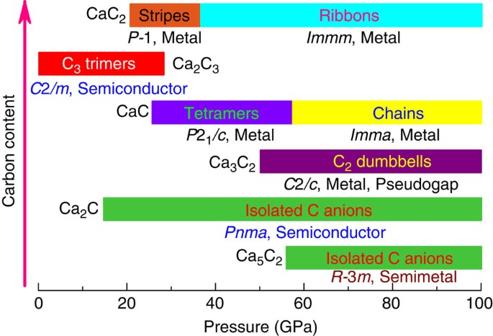Figure 4: Carbon arrangement with increasing carbon content. Only thermodynamically stable phases are shown (For metastable phases, seeSupplementary Table 2). Additionally, the conducting properties are shown. Full size image Figure 4: Carbon arrangement with increasing carbon content. Only thermodynamically stable phases are shown (For metastable phases, see Supplementary Table 2 ). Additionally, the conducting properties are shown. Full size image Ca 5 C 2 The stable structure of Ca 5 C 2 has a R -3 m symmetry. It is a semi-metal (see Supplementary Fig. 8 ) and is thermodynamically stable at pressures ranging from 58 GPa to at least 100 GPa (see Fig. 4 ). This phase has novel structural features: it can be described as consisting of alternating CaC 2 layers (where Ca is octahedrally coordinated by C atoms) and layers with composition Ca 4 . The electron localization function distribution in Ca 5 C 2 shows strong charge transfer from Ca to C. Non-nuclear charge density maxima are located in the Ca 4 layer as plotted in Fig. 5 (electron localization function=0.75 at 60 GPa). Bader charges are +1.039 for Ca1, +0.823 for Ca2, +0.973 for Ca3 and −0.459 for the interstitial electron density maximum. 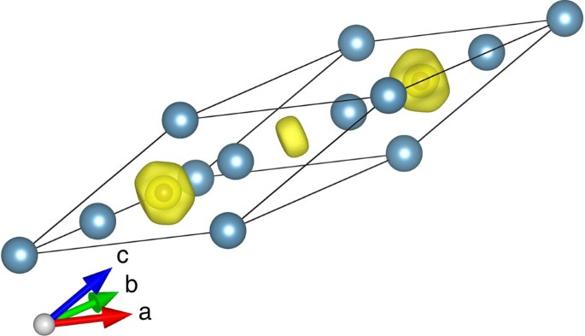Figure 5: Electron localization function (ELF) ofR-3m-Ca5C2at 60 GPa. The isosurface ELF=0.75 is shown. The observed interstitial electron charge accumulation shows that Ca5C2withR-3msymmetry is an electride. Figure 5: Electron localization function (ELF) of R -3 m -Ca 5 C 2 at 60 GPa. The isosurface ELF=0.75 is shown. The observed interstitial electron charge accumulation shows that Ca 5 C 2 with R -3 m symmetry is an electride. Full size image Ca 2 C Known alkali earth methanides include well-know Be 2 C ( Fm -3 m , Z=4) and Mg 2 C (antifluorite) recently synthesized by Kurakevych et al . [25] However, no theoretical or experimental information has been reported on the methanide Ca 2 C (ref. 26 ). According to our calculations, Ca 2 C is thermodynamically stable above 15 GPa (space group Pnma (Z=4)). For Pnma -Ca 2 C we observe the largest negative charge of carbon atoms among all these phases: −2.321. In this semiconducting phase with band gap of 0.64 eV at 14 GPa (see Supplementary Fig. 9 ), C atoms are isolated and one can represent this compound as a carbide with an idealized charge transfer scheme (Ca 2+ ) 2 C 4− adhering to the Zintl concept. Metallic metastable C 2 /m -Ca 2 C has a unique structure, consisting of alternating layers of stoichiometry Ca 2 (C 2 ) and Ca 2 (two kinds of calcium atoms play distinctly different roles, see Fig. 6 a ), and these layers have net charges of +0.582 and −0.582, respectively (see Supplementary Table 1 ). What is unusual is that the Ca layer is negatively charged, that is, it is a reservoir of electrons. To further analyse this phenomenon, it is instructive to look first at the Ca 2 (C 2 ) layer. This C 2 group can be represented as having a triple C–C bond and its ideal charge is −2 (Bader charge is −1.892), and if each Ca had the ideal charge of +2, the total charge of the Ca 2 (C 2 ) layer would be +2, and two electrons would be transferred to the Ca 2 layer (see Supplementary Table 1 ). In reality, the C–C bond here has a somewhat lower order (C–C distance is 1.28 Å at 5 GPa) and therefore takes more electrons from Ca atoms, leaving less for the Ca 2 layer, but not changing the picture qualitatively. To our knowledge, this is the first example of negatively charged metal atoms in a compound with more electronegative atoms. Note the enormous difference of Bader volumes of the positively and negatively charged Ca atoms (16.570 versus 41.901 Å 3 ). One can expect that the electrons in the Ca layer are very loosely bound, and the work function of this compound can be expected to be extremely low. The density of states of the metastable C 2 /m phase of Ca 2 C reveals a remarkable step-like feature near the bottom of the valence band, followed by a nearly constant density of states (see Fig. 6b ), presenting an example of a quasi-2D electronic structure as observed in Li–Be alloys [27] . The calculated Fermi surface of C 2 /m -Ca 2 C at 3 GPa has a hollow square cylinder-like Fermi shape along the Γ-V direction (that is, reciprocal lattice basis vector b 3 direction) in the Brillouin zone (BZ), signalling quasi-2D electronic properties (see Fig. 6c ). 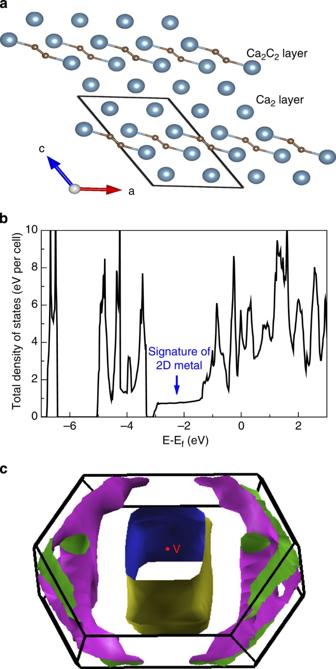Figure 6: Structural and electronic property ofC2/mphase of Ca2C at 3 GPa. (a) The top view ofC2/mstructure along the y axis shows a clearly layered structure. (b)Total electronic density of states (DOS). (c) Fermi surface of theC2/mstructure. The indication of a quasi-two-dimensional metal in total DOS is confirmed by the hollow square prismatic cylinder-like Fermi surface. Figure 6: Structural and electronic property of C 2 /m phase of Ca 2 C at 3 GPa. ( a ) The top view of C 2 /m structure along the y axis shows a clearly layered structure. ( b )Total electronic density of states (DOS). ( c ) Fermi surface of the C 2/ m structure. The indication of a quasi-two-dimensional metal in total DOS is confirmed by the hollow square prismatic cylinder-like Fermi surface. Full size image Ca 3 C 2 For Ca 3 C 2 , no thermodynamically stable phase exists below 50 GPa. A metastable P 4 /mbm (Z=2) phase, favoured in the pressure range from 5 to 30 GPa, transforms into a C 2 /c (Z=4) structure at 30 GPa, which is thermodynamically stable above 50 GPa. The structure of P 4 /mbm -Ca 3 C 2 contains doubly bonded C 2 groups (C–C distance 1.39 Å at 20 GPa), with an ideal charge −4, that is, accepting four electrons from calcium atoms, leaving two electrons per formula to form Ca–Ca bonds in this metallic compound. Metallic C 2 /c -Ca 3 C 2 with a pseudogap at the Fermi level (see Supplementary Fig. 10 ) has singly bonded C 2 groups (C–C bond length 1.51 Å at 38.7 GPa), which have ideal charge −6, exactly balanced by three Ca atoms in the formula. CaC Metallic CaC has two thermodynamically stable phases below 100 GPa. At 14 GPa, the metastable orthorhombic Immm structure transforms into a monoclinic P 2 1 / c structure (stable thermodynamically above 26 GPa, favoured over a wide pressure range of 14–57.5 GPa), followed by a thermodynamically stable Imma structure. P 2 1 /c -CaC is very interesting because its structural formula Ca 4 (C 4 ) contains a unique and hitherto unknown zigzag C 4 group, with C–C distances between 1.48 and 1.50 Å at 14 GPa, indicating bond orders between 1 and 2 and ideal charges of about −2.5 for the end C atoms (Bader charge −1.447) and about −1 for the central C atoms (Bader charge −0.905). Imma -CaC has infinite zigzag chains of C atoms (C–C bond length of 1.55 Å at 57.5 GPa, indicating a weakened single bond) in the y axis direction. The structural formula of metastable Immm -CaC is Ca 2 (C 2 ), and with a doubly bonded C 2 group (C–C distance 1.33 Å at 7.1 GPa) that has an ideal charge of −4 (Bader charge –2.340), it exactly balances the ideal charge of two Ca atoms. All three phases of CaC beautifully conform to the trend of increasing polymerization of the C sublattice with increasing pressure. Ca 2 C 3 The structure of Mg 2 C 3 (space group Pnnm , Z =2), the only known alkaline-earth metal allylenide with C 3 4− anions [26] , was considered when searching for stable phases of Ca 2 C 3 . Total energy calculations exclude the possibility of the ambient-pressure Mg 2 C 3 -type structure. The semiconducting C 2 /m structure (band gap of 1.06 eV at 10 GPa, see Supplementary Fig. 11 ) is instead the most stable one below 34.5 GPa (thermodynamically stable from 0 to 28 GPa), followed by metastable C 2 /c structure. By fitting energy versus volume data to the third-order Birch–Murnaghan equation of state [28] , the calculated bulk modulus B 0 of C 2 /m -Ca 2 C 3 is ∼ 89 GPa, which is higher than that of CaC 2 (50 GPa). At ∼ 40 GPa, the metallic C 2 /c structure transforms into a metastable P -1 structure (metal), which dominates the pressure range between 40 and 65 GPa. At higher pressures, a metallic metastable Imma structure is stable and contains zigzag carbon chains ( Figs 3 and 4 ). We searched at much higher pressures for 3D-polymeric carbon frameworks in Ca 2 C 3 , but found none at pressures up to at least 300 GPa. For comparison, in CaC 2 we have found that graphene sheets predicted in the high-pressure phase can be stable up to at least 1 TPa (ref. 16 ). For Ca 2 C 3 , the carbon arrangement changes from isolated C 3 to carbon chains to ribbons ( Fig. 3 ). The structure of C 2 /m -Ca 2 C 3 can be described as Ca 2 layers linked together by nearly linear symmetric C 3 groups with double C–C bonds (C–C distances 1.32 Å at 18.1 GPa). With this configuration, the total charge of the C 3 group should be −4 (Bader charge −2.692), exactly compensating the charge of two Ca atoms in the formula (see Supplementary Table 1 ). Central carbon atoms in the C 3 group in this valence scheme should be neutral, and yet turn out to have a large negative Bader charge of −0.738, whereas the end atoms, whose idealized charge is −2, develop a lower Bader charge (−0.977). This discrepancy is explained by the effects of Ca atoms, which form significant bonds with the central carbon atom in the C 3 group and transfer some electronic charge to them. Most recently, some of us reported the prediction and synthesis of β-Mg 2 C 3 (ref. 29 ), which is isostructural with our C 2 /m -Ca 2 C 3 reported here. The structure of C 2 /c -Ca 2 C 3 (C–C distances 1.43–1.47 Å at 34.5 GPa) has an idealized charge transfer scheme Ca 2 4+ C 3 4− . In this metallic phase, C atoms are polymerized into infinite chains with nearly closed six-member rings running through channels of Ca host lattice. P -1-Ca 2 C 3 features a complicated extended 1D ribbon of carbon atoms with nearly single C–C bonds (lengths 1.47–1.50 Å at 40 GPa). Imma -Ca 2 C 3 has a very interesting structure with extended 1D ribbons of carbon atoms cut from the graphene layer. Bond lengths in this ribbon are 1.50–1.52 Å at 70 GPa, slightly longer than in graphene and indicating predominantly single bonds. Electronic structure calculations show that both P -1 and Imma phases of Ca 2 C 3 are metals. On the basis of Allen and Dynes modified equation [30] , we have checked for superconductivity in these phases at 34 and 65 GPa, respectively, and found none. CaC 2 CaC 2 is thermodynamically stable above 21 GPa (see Fig. 1a ). The lower-pressure phases C 2 /m and Cmcm reported previously [16] are metastable, which could be unravelled by calculating enthalpy of formation (Δ H f ) at lower pressure. Considering that graphite is the ground state of carbon at zero pressure, we performed additional calculations where the van der Waals interaction is accounted for by using the optPBE-van der Waals functional [31] . At zero pressure, the calculated Δ H f (−0.17 eV per atom) of CaC 2 is close to the experimental standard Δ H f (−0.21 eV per atom at 298 K and 1 atm (ref. 32 )) but higher than that (−0.27 eV) of Ca 2 C 3 , confirming the thermodynamic metastability of CaC 2 under ambient conditions (see Fig. 1a ). It is very unexpected, but the above numbers fully confirm this conclusion, that the well-known and industrially produced compound CaC 2 is metastable under ambient conditions, while the so far never seen compound Ca 2 C 3 is actually stable. This could be either due to kinetics, or due to high-temperature conditions of synthesis. In addition to our previous result [16] , we found a new phase with the P -1 symmetry, which contains infinite carbon chains with five-membered rings (C–C distance is between 1.442 and 1.507 Å at 20 GPa (see Fig. 3i ), signalling single or double bonds), and is the lowest enthalpy structure over a wide pressure range from 7.5 to 37 GPa (thermodynamically stable from 21 to 37 GPa, see Fig. 4 and Supplementary Fig. 12 ). With further application of pressure, metallic P -1-CaC 2 transforms into metallic Immm -CaC 2 (ref. 16 ), in which carbon atoms are polymerized to form quasi-1D ribbons (see Figs 2 , 3 ). Experiments In order to confirm theoretical structure predictions, we performed synthesis under high-pressure/high-temperature conditions. Diamond anvil cells were loaded with both calcium- and carbon-rich Ca+C mixtures, compressed to pressures up to 25 GPa, heated to temperatures up to ∼ 2,000 K and probed in situ using synchrotron PXRD. Under these pressure conditions, the formation of Immm -CaC 2 , C 2 /m -Ca 2 C 3 and Pnma -Ca 2 C may be expected on the basis of thermodynamic stabilities, as these phases are the only stable ones that appear on the convex hull up to 25 GPa (see Fig. 1 ); indeed, two of these three structures were observed experimentally. When samples were compressed above ∼ 10 GPa and heated to ∼ 2,000 K, mixtures of elemental glassy carbon and face-centred cubic ( fcc ) Ca transformed into a new low-symmetry phase. After comparison with density functional theory (DFT) structure predictions, PXRD reflections originating from this phase were readily indexed to the monoclinic C 2 /m -Ca 2 C 3 structure with excellent agreement between experiment and theory (see Supplementary Table 3 ). 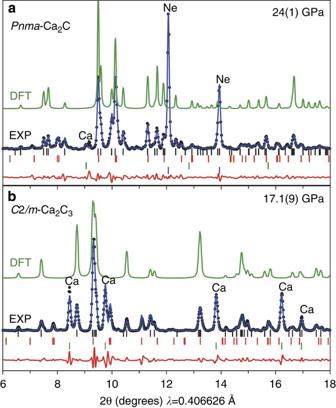Figure 7: PXRD patterns for experimentally observed Ca-C phases. (a)Pnma-Ca2C synthesized at 24 GPa (wRp=1.5%,Rp=0.9%). (b)C2/m-Ca2C3synthesized at 17 GPa (wRp=2.0%,Rp=0.9%). Experimental data (points) are compared with full-profile refinements using the Le Bail method (blue lines), with differences (red lines). Simulated powder patterns using atomic positions derived from DFT-optimized structures are shown for intensity comparison (green lines). Positions of reflections of Ca2C (a) or Ca2C3(b), Ca, Ne and a third carbide phase (seeSupplementary Note 2) are indicated by black, green, blue and red tick marks, respectively. Figure 7 shows experimental PXRD data obtained at 17 GPa with a =5.169(4) Å, b =4.994(3) Å, c =6.322(3) Å and β =128.53(3)°, which compares with a =5.151 Å, b =4.962 Å, c =6.306 Å and β =128.81° for the theoretical structure relaxed at 18 GPa. This sample was decompressed in steps of ∼ 2 GPa to obtain lattice parameters as a function of pressure (see Fig. 8 ). Theoretical lattice parameters show an average absolute deviation of 0.3% from experiment over the entire pressure range, and the C 2 /m -Ca 2 C 3 phase was recoverable to ambient pressure, but was found to be air/moisture-sensitive. The experimental P–V data were fit to a second-order Birch–Murnaghan equation of state with B 0 =84(2) GPa, in good agreement with theoretical predictions (89 GPa). Figure 7: PXRD patterns for experimentally observed Ca-C phases. ( a ) Pnma -Ca 2 C synthesized at 24 GPa ( wR p =1.5%, R p =0.9%). ( b ) C 2 /m -Ca 2 C 3 synthesized at 17 GPa ( wR p =2.0%, R p =0.9%). Experimental data (points) are compared with full-profile refinements using the Le Bail method (blue lines), with differences (red lines). Simulated powder patterns using atomic positions derived from DFT-optimized structures are shown for intensity comparison (green lines). Positions of reflections of Ca 2 C ( a ) or Ca 2 C 3 ( b ), Ca, Ne and a third carbide phase (see Supplementary Note 2 ) are indicated by black, green, blue and red tick marks, respectively. 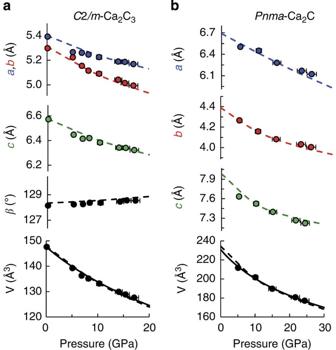Figure 8: Lattice parameters and unit cell volumes for Ca-C phases. Experimental parameters (points) are compared with DFT predictions (dashed lines) for bothC2/m-Ca2C3(a) andPnma-Ca2C (b). Experimentally-derived equations of state for both phases are shown as solid lines in the lower panels. Full size image Figure 8: Lattice parameters and unit cell volumes for Ca-C phases. Experimental parameters (points) are compared with DFT predictions (dashed lines) for both C 2 /m -Ca 2 C 3 ( a ) and Pnma -Ca 2 C ( b ). Experimentally-derived equations of state for both phases are shown as solid lines in the lower panels. Full size image At pressures above ∼ 22 GPa, a second carbide phase ( Pnma -Ca 2 C) was synthesized upon laser heating. This same phase was reproducibly formed both from elemental Ca+C mixtures and from samples containing C 2 /m -Ca 2 C 3 , indicating disproportionation of Ca 2 C 3 into a more stable carbide phase when pressure is raised above ∼ 22 GPa, i.e. above its predicted stability field. Figure 7 shows experimental PXRD data at 24 GPa with a =6.122(1) Å, b =4.004(1) Å, c =7.223(1) Å, which compares with a =6.044 Å, b =3.977 Å, c =7.265 Å for DFT calculations at the same pressure (see Supplementary Table 4 ). Calculated lattice parameters show an average absolute deviation of 0.5% from experimental values between 25 and 5 GPa (see Fig. 8 ), which was the lowest pressure obtained due to failure of a diamond anvil. Fitting the P–V data to a second-order Birch–Murnaghan equation of state yields B 0 =53(4) GPa. We find that the carbon sublattice within all predicted carbide phases has close correlation with the Ca:C ratio (see Fig. 2 ). With increasing carbon content, isolated carbon atoms are polymerized, in turn, into C 2 dumbbells, C 3 and C 4 groups, chains, ribbons and graphene sheets (see Fig. 4 and Supplementary Table 2 ). The polymeric carbon structures reveal an expected trend when comparing with the structural chemistry of the heavier congeners of group IV elements in Zintl phases (alkali or alkaline-earth silicides, germanides and stannides) [17] , [33] . Yet in spite of certain similarities to silicides, calcium carbides differ from them because of distinct bonding features. Combining present analysis and our previous results [16] , [17] , [20] , one can conclude that for the Ca-C system, one can cover sp to sp 2 to sp 2 + sp 3 to sp 3 hybridizations of carbon as pressure increases. This pressure-induced structural evolution of carbon was also found in other alkali metal or alkaline-earth metal carbides [17] , [20] , [24] . Together with our previous results for CaC 2 (ref. 16 ) and CaC 6 (ref. 20 ), it is clear that a 3D network of carbon in CaC x can be formed when x is greater than 2 (from sheets to 3D frameworks to Ca-C phase separation with slabs of diamond at high C content), consistent also with the behaviour of the metastable CaC 4 compound found in our structural searches. On the other hand, the structural features of carbon-rich compounds [20] can be extended to alkali-metal or alkaline-earth metal congeners of the group-IV elements, which allows one to fabricate a variety of the 3D framework structures of the group-IV elements by removing metal sublattices. The unexpected mechanical [20] , [34] or electronic characteristics [35] uncovered in these 3D framework structures pave the way to novel materials. In summary, we have produced the first complete pressure-composition phase diagram for CaC x compounds at pressures up to 100 GPa and demonstrated the experimental synthesis of two previously unknown compounds (Ca 2 C 3 and Ca 2 C), validating part of our predicted phase diagram. Contrary to normal ionic compounds, there is no ‘dominant’ compound stable in this whole pressure range. The well-known CaC 2 and CaC 6 were found to be metastable at normal conditions; CaC 2 is stable only above 21 GPa, and CaC 6 is never thermodynamically stable, while hitherto unreported Ca 2 C 3 is actually thermodynamically stable at ambient pressure. Bader analysis unravels very diverse chemistry: the decrease in C–C bond order from triple to double to single bonds at increasing pressure; a negatively charged metal layer in calcium-rich Ca 2 C compound; a hitherto unknown bent linear C 4 group in the P 2 1 / c phase of CaC; C ribbons being present in carbon-rich compounds. The C 2/ m -Ca 2 C phase provides a fresh and very attractive example of a 2D metal, presenting the only known example of a compound where a metal atom (Ca) develops a negative Bader charge in presence of a more electronegative atom (C). Such unusual compounds are likely to find potential applications if synthesized in sufficiently large quantities. While powerful computational methods, such as USPEX, are capable of reliably predicting these exotic compounds, simple theoretical models capable of anticipating them are yet to be developed. Structure search and theoretical calculations Searches for stable structures of the Ca-C system under compression were carried out using the evolutionary algorithm USPEX in combination with the VASP code [36] on the basis of DFT within the generalized gradient approximation with the exchange-correlation functional of Perdew, Burke and Ernzerhof [37] , employing the projector-augmented wave [38] method [He] and [Ne] cores for C and Ca atoms, respectively. For carbon, a ‘hard’ PAW potential was used in search for stable structures. For the crystal structure searches, we used a plane-wave basis set cutoff of 700 eV and performed the BZ integrations using uniform Gamma-centred k-point meshes. The most interesting structures were further relaxed at a higher level of accuracy with a basis set cutoff of 1,000 eV and a k-point grid of spacing 2 π × 0.018 Å −1 . Iterative relaxation of atomic positions was stopped when all forces were smaller than 0.001 eV Å −1 . For compounds predicted via variable-composition searches, we re-searched their stable structures using fixed-composition calculations, with two, three and four formula units per unit cell. For Ca 2 C 3 , some evolutionary calculations were also performed under the pressure of 30, 50, 80, 120, 160, 240 and 300 GPa with two or four chemical formula units per unit cell so as to discern the possibility of 3D network carbon. The enthalpy of formation per atom of Ca n C m is defined as Δ H f (Ca n C m )=[ H (Ca n C m )- nH (Ca)- mH (C)]/( n + m ), where all enthalpies H are given at the same pressure and zero temperature. At a given pressure, the calcium carbides located on the convex hull are thermodynamically stable against decomposition to any other binaries or the elements, while the compounds above the convex hull are meta-stable. The Bader analysis was performed for exploring chemical bonding and local electrons [39] . To get a converged charge density, the plane wave kinetic energy cutoff of 1,000 eV and Monkhorst-Pack k -point meshes with the reciprocal space resolution of 2 π × 0.02 Å −1 were used for all the structures. A series of FFT grids to accurately reproduce the correct total core charge were tested by increasing parameters NG(X,Y,Z)F to 1.5, 2 and 2.5 times the default one. The lattice dynamics and superconducting properties of Ca 2 C 3 were calculated by the Quantum ESPRESSO package [40] using Vanderbilt-type ultrasoft pseudopotentials with cutoff energies of 50 and 500 Ry for the wave functions and the charge density, respectively. The electronic BZ integration in the phonon calculation was based on a 12 × 12 × 12 of Monkhorst-Pack k-point meshes. The dynamical matrix was computed on the basis of a 6 × 6 × 6 mesh of phonon wave vectors. The electron–phonon coupling was convergent with a finer grid of 48 × 48 × 48 k points and a Gaussian smearing of 0.01 Ry. For other compounds, phonon calculations were performed using the Phonopy code [41] . The Fermi surface of C 2 /m -Ca 2 C at 3 GPa was calculated using Quantum Espresso and 16 × 16 × 8 of Monkhorst-Pack k-point mesh. Experiment Reagents for experimental studies consisted of commercial calcium metal (Sigma-Aldrich, dendritic pieces, 99.99%) and glassy carbon (Sigma-Aldrich, 2–12 μm, 99.95%). The carbon powder was degasified for 12 h at ∼ 200 °C in a vacuum oven and then sealed under Ar. Diamond anvil cell syntheses (up to 25 GPa and 2,000 K with in situ PXRD) were performed at High Pressure Collaborative Access Team (HPCAT), sector 16, of the Advanced photon Source. A small amount of carbon powder and Ca metal shavings were pressed in thin layers within a rhenium gasket in a diamond anvil cell equipped with 400-μm culet diamonds inside of an inert Ar glovebox (O 2 <1 p.p.m. ; H 2 O<1 p.p.m.). It was not possible to control the precise Ca:C ratio; however, compositions were estimated to range between 0.333≤Ca:C≤3, on the basis of the volume of material loaded into the diamond cell. Samples were sealed inside the glovebox without pressure medium or loaded with Ne to improve thermal isolation from diamonds and quasi-hydrostatic conditions for subsequent diffraction measurements. Pressure was estimated using the Ne equation of state [42] and/or with a ruby gauge [43] . To generate high temperatures, samples were heated on both sides using infrared fibre lasers. In some cases two or three heating cycles were performed, with X-ray diffraction patterns collected before, during and after laser heating. During laser heating, temperatures from each side of the sample were estimated by collecting emitted thermal radiation, correcting for the optical system response and fitting the spectral data to Planck’s equation. Angle-dispersive PXRD patterns were collected using a mar345 detector (marXperts GmbH, Norderstedt, Germany) image plate calibrated with a CeO 2 standard. Patterns were integrated using FIT2D (ref. 44 ) and phase recognition and indexing were performed using PowderCell and CheckCell programmes [45] . While observed PXRD intensities were in good agreement with DFT-derived structural models, observed powder statistics were not suitable for Rietveld refinements. Full profile refinements were performed using the Le Bail intensity extraction method, as implemented in GSAS [46] with EXPGUI [47] (see Supplementary Figs 13–15 and Supplementary Note 2 for additional details). How to cite this article : Li, Y. L. et al . Investigation of exotic stable calcium carbides using theory and experiment. Nat. Commun . 6:6974 doi: 10.1038/ncomms7974 (2015).